Whole-genome mutational landscape of liver cancers displaying biliary phenotype reveals hepatitis impact and molecular diversity Intrahepatic cholangiocarcinoma and combined hepatocellular cholangiocarcinoma show varying degrees of biliary epithelial differentiation, which can be defined as liver cancer displaying biliary phenotype (LCB). LCB is second in the incidence for liver cancers with and without chronic hepatitis background and more aggressive than hepatocellular carcinoma (HCC). To gain insight into its molecular alterations, we performed whole-genome sequencing analysis on 30 LCBs. Here we show, the genome-wide substitution patterns of LCBs developed in chronic hepatitis livers overlapped with those of 60 HCCs, whereas those of hepatitis-negative LCBs diverged. The subsequent validation study on 68 LCBs identified recurrent mutations in TERT promoter, chromatin regulators ( BAP1 , PBRM1 and ARID2 ), a synapse organization gene ( PCLO ), IDH genes and KRAS . The frequencies of KRAS and IDHs mutations, which are associated with poor disease-free survival, were significantly higher in hepatitis-negative LCBs. This study reveals the strong impact of chronic hepatitis on the mutational landscape in liver cancer and the genetic diversity among LCBs. Primary liver cancer is the fifth most common cancer and the third leading cause of cancer death worldwide. Virus infection is the most common and strongest aetiological factor for liver cancer development. Pathologically, primary liver cancer can be classified into ~90% hepatocellular carcinoma (HCC), and 5~10% intrahepatic cholangiocarcinoma (ICC), and the combined hepatocellular cholangiocarcinoma (cHCC/CC), representing only a small portion [1] , [2] , [3] . Clinically, ICC and cHCC/CC show much more aggressive behaviour with poorer prognosis than HCC, and no standard treatment currently exists, other than surgical resection [1] . One of the major risk factors for the development of ICC is chronic inflammation of the bile ducts, including chronic infections caused by biliary flukes, primary sclerosing cholangitis and hepatolithiasis [2] , [4] . Furthermore, recent epidemiological studies recognized that chronic hepatitis associated with viral infection (hepatitis B virus (HBV) and hepatitis C virus (HCV)) is also an important aetiologic factor of ICC, as well as HCC, in Asia [2] , and indicated that hepatitis-associated ICC and HCC share a common disease process for carcinogenesis [5] . HCC and ICC have been reported to develop simultaneously in both human and mouse models [5] , [6] , [7] and a combined or mixed phenotype (cHCC/CC) displays intimately mixed components of both hepatocellular and biliary epithelial differentiation [8] , as shown in Fig. 1a . The presence of these phenotypes indicates the possibility that some of liver cancers can arise from liver progenitor or liver stem cell, although exact cell origins of ICC and cHCC/CC are still controversial and remain to be elucidated [6] , [9] . We here define ICC and cHCC/CC, both of which contain varying degrees of biliary epithelial differentiated cells, as liver cancer displaying biliary phenotype (LCB), distinguishing from HCC phenotype ( Fig. 1a ). Although several genome analyses of HCC and exome studies of ICC have been recently reported [10] , [11] , [12] , [13] , [14] , [15] , [16] , [17] , [18] , [19] , [20] , the whole-genomic aberration signature of LCB and its comparison with HCC has yet to be comprehensively explored. In addition, the influence of aetiological factors, such as chronic hepatitis and virus infection type, on the mutational landscape of primary liver cancer remains unknown and has just begun to be analyzed [21] . 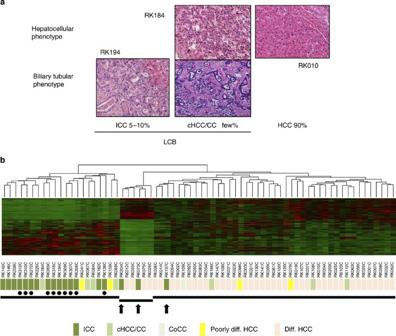Figure 1: LCB phenotype and analysis of the transcriptome pattern on the 30 LCBs and 60 HCCs. (a) Representative pathological images of ICC, cHCC/CC and HCC. RK194 is intrahepatic well-differentiated cholangiocarcinoma. RK184 is cHCC/CC where some sections show moderately or poorly differentiated cholangiocarcinoma (lower) and some show moderately differentiated HCC (upper). RK010 is moderately differentiated HCC. We define ICC and cHCC/CC, both of which contain varying degrees of biliary tubular-differentiated cells, as liver cancer displaying biliary phenotype (LCB), distinguishing from HCC phenotype. (b) Clustering by the transcriptome of 25 LCBs and 44 HCCs. Hepatitis-negative LCBs are indicated by black dots. ICC, cHCC/CC, CoCC (cholangiolocellular carcinoma), poorly differentiated HCC and differentiated HCC are indicated by coloured rectangles. Three ICCs with metachronous MCTs of HCC are indicated by arrows. Figure 1: LCB phenotype and analysis of the transcriptome pattern on the 30 LCBs and 60 HCCs. ( a ) Representative pathological images of ICC, cHCC/CC and HCC. RK194 is intrahepatic well-differentiated cholangiocarcinoma. RK184 is cHCC/CC where some sections show moderately or poorly differentiated cholangiocarcinoma (lower) and some show moderately differentiated HCC (upper). RK010 is moderately differentiated HCC. We define ICC and cHCC/CC, both of which contain varying degrees of biliary tubular-differentiated cells, as liver cancer displaying biliary phenotype (LCB), distinguishing from HCC phenotype. ( b ) Clustering by the transcriptome of 25 LCBs and 44 HCCs. Hepatitis-negative LCBs are indicated by black dots. ICC, cHCC/CC, CoCC (cholangiolocellular carcinoma), poorly differentiated HCC and differentiated HCC are indicated by coloured rectangles. Three ICCs with metachronous MCTs of HCC are indicated by arrows. Full size image To elucidate the molecular features of these liver cancer phenotypes, we compared whole-genome sequencing (WGS) data of 30 LCBs and 60 HCCs, and RNA sequencing data for 25 LCBs and 60 HCCs. We examine the WGS to elucidate the substitution pattern and identify driver genes. Finally, we investigate the tumour heterogeneity to find the genes with clonal mutations by target deep-sequencing analysis. This study demonstrates the first genome-wide comparison of LCBs with and without chronic hepatitis and characterizes their molecular features. Samples and WGS In this study, frozen tumour and matched normal tissues were collected from 30 patients with LCB ( Table 1 ) and 60 patients with HCC ( Supplementary Table 1 ). All samples were used for WGS. RNA from 25 LCB and 44 HCC samples, from which high-quality RNA was obtained, was also sequenced. Of the LCB samples, 21 were pathologically classified as typical ICC, 2 as rare type of ICC, cholangiocellular carcinoma (CoCC) and 7 as cHCC/CC. Epidemiologically, 9 were from a HCV-related hepatitis background, 7 from HBV-related hepatitis and 14 were not infected with HBV nor HCV. Among them, 10 cases had normal livers with no pathological feature of chronic hepatitis and fibrosis. RK204 (ICC) and RK209 (HCC) developed metachronously in a single individual as multicentric tumours. 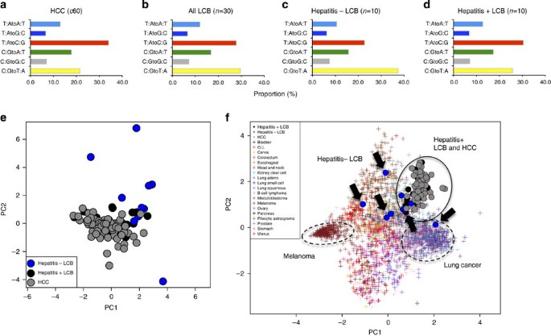Figure 2: Genome-wide substitution pattern on the 30 LCBs and 60 HCCs. Average proportion of somatic nucleotide substitutions for (a) the 60 HCCs, (b) the 30 LCBs, (c) the 10 hepatitis-negative LCBs and (d) the 20 hepatitis-positive LCBs. (e) Principal component analysis (PCA) of the whole-genome substitution patterns of the 30 LCBs and 60 HCCs. Hepatitis-positive LCBs (black dots) overlap the HCC cluster (gray). LCBs developed in livers without hepatitis (blue dots) diverged from others. (f) PCA of the whole-genome substitution patterns of the 30 LCBs, the 60 HCCs and other types of cancers21. Hepatitis-positive liver cancers (HCC and LCBs) are tightly clustered, as are melanomas, indicating that chronic hepatitis or inflammation can strongly impact the somatic mutation signature. Genomic DNA was extracted from the tumour and matched lymphocyte or non-tumour liver samples, and WGS was performed at 40.0x average coverage for tumour samples and 33.0x for matched normal tissue, after removing polymerase chain reaction (PCR) duplicates ( Supplementary Table 2 ). For comparison, we used the somatic mutation data of the 60 HCCs that have been whole-genome sequenced by RIKEN and deposited to the ICGC dataset version 8 released on 2012 March ( https://dcc.icgc.org/ ). Table 1 Clinical and pathological features of 30 LCBs analyzed by whole-genome sequencing. Full size table Whole-genome mutational landscape of LCBs We identified point mutations, short indels, copy number alternations, HBV integration sites and somatic rearrangements using custom algorithms (see Methods). We detected between 345 and 180,117 point mutations per tumour. RK308 had an exceptionally large number of somatic mutations (180,117 point mutations), exhibiting a DNA mismatch-repair deficiency with a homozygous deletion in the MLH1 gene and a missense mutation (C199R) in the MSH2 gene, which was previously found in Lynch syndrome patient with DNA mismatch-repair deficiency and proved to disrupt its function [22] . Excluding RK308, the average number of nonsynonymous mutations in the 29 LCBs was 26.2, larger than previously reported for leukaemia, but lower than for HCC, lung cancer and melanoma [23] ( Supplementary Fig. 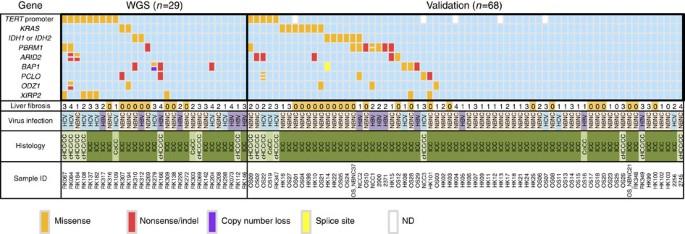Figure 3: Analysis of recurrently mutated genes in LCBs. Recurrently mutated genes in the 30 LCB WGS set and the 68 validation LCB set. Histological subtype of LCB: ICC; intrahepatic cholangiocarcinoma, cHCC/CC; combined hepatocellular-cholangiocarcinoma and CoCC; cholangiolocellular carcinoma. Liver fibrosis was determined according to the New Inuyama Classification (0~4). Liver fibrosis 0 indicates hepatitis-negative LCB. Virus infection status is classified as HBV, HCV or negative, which was determined by serological study. 1 , and Supplementary Table 3 ). The number of detected somatic rearrangements varied greatly among samples (0–260) ( Supplementary Fig. 2 and Supplementary Dataset 1 ). Chromothripsis was observed in RK142 and RK316 ( Supplementary Fig. 2j and 2ac ). HBV integration sites were identified in three LCBs (RK069:cHCC/CC, RK166:cHCC/CC, RK208:ICC) using read-pair information [12] , [14] , [15] ( Supplementary Table 4 and Supplementary Methods ), indicating that HBV-infection and its genomic integration can be involved with the carcinogenesis of LCBs [24] , [25] . Gene expression patterns of LCBs and HCCs To gain molecular insight into the differences between LCBs and HCCs, we examined their gene expression profiles ( Fig. 1b ). RNA-seq analysis on 25 LCBs and 44 HCCs, whose high-quality RNAs were available among the 30 LCBs and 60 HCCs, clustered most LCBs into one group, along with some poorly differentiated HCCs, suggesting that LCBs may be similar to poorly differentiated HCCs ( Fig. 1b ) and that LCBs may have some progenitor feature similar to poorly differentiated HCCs [7] . Some cHCC/CCs clustered in the LCB group, whereas others were in the main HCC group, which is consistent with their histological combined features. Interestingly, three ICCs with HCC metachronous multicentric tumours were classified within the HCC group (RK204, RK073 and RK137). One CoCC was clustered in the HCC group, which suggests that this particular liver tumour may have an origin similar to that of cHCC/CC [26] . Somatic substitution pattern of LCB and HCC Next we examined somatic substitution patterns of LCBs and compared with those of 60 HCCs ( Fig. 2a–d ). The distribution of genome-wide somatic substitution patterns is significantly different from random expectation ( χ 2 -test; P- value<10 −16 ). In the LCB genomes, the most predominant substitution was C:G to T:A (odds ratio=2.2, comparison from the assumption of the uniform mutation rate), followed by T:A to C:G (odds ratio=1.9) and C:G to A:T (odds ratio=1.3) ( Fig. 2b ). The distribution of the substitution pattern for LCBs and HCCs was similar ( Fig. 2a,b ), but the proportion of C:G to T:A was significantly higher in LCBs ( Supplementary Fig. 3 ). To examine the differences between each sample, principal component analysis (PCA) was applied to the somatic substitution patterns. Although most LCB somatic substitution patterns overlapped the 60 HCC cluster, those of the eight LCBs, all of which developed in livers with no evidence of chronic hepatitis, diverged ( Fig. 2e and Supplementary Fig. 4 ). To compare the difference between the HCCs, the hepatitis-positive LCBs and the hepatitis-negative LCBs in the PCA, we performed a permutation test. The difference between the hepatitis-positive and -negative LCBs, and between the hepatitis-negative LCBs and the HCCs were significantly larger than those from randomly selected samples after the Bonferroni correction (hepatitis-positive and negative LCBs; P- value=0.00116, and the hepatitis-negative LCBs and the HCCs; P- value < 0.00001). Figure 2: Genome-wide substitution pattern on the 30 LCBs and 60 HCCs. Average proportion of somatic nucleotide substitutions for ( a ) the 60 HCCs, ( b ) the 30 LCBs, ( c ) the 10 hepatitis-negative LCBs and ( d ) the 20 hepatitis-positive LCBs. ( e ) Principal component analysis (PCA) of the whole-genome substitution patterns of the 30 LCBs and 60 HCCs. Hepatitis-positive LCBs (black dots) overlap the HCC cluster (gray). LCBs developed in livers without hepatitis (blue dots) diverged from others. ( f ) PCA of the whole-genome substitution patterns of the 30 LCBs, the 60 HCCs and other types of cancers [21] . Hepatitis-positive liver cancers (HCC and LCBs) are tightly clustered, as are melanomas, indicating that chronic hepatitis or inflammation can strongly impact the somatic mutation signature. Full size image To compare the impact of chronic hepatitis and inflammation on the somatic substitution pattern, we performed PCA with several types of cancer [21] . In the PCA plot, cancers strongly influenced by specific mutagens, such as melanoma (UV-exposure) and lung cancer (smoking), were tightly clustered, suggesting that a strong impact of these mutagen exposures on substitution patterns causes a reduction in the divergence among the samples ( Fig. 2f ). The HCCs, most of which were associated with chronic hepatitis, and the hepatitis-positive LCBs tightly clustered together, whereas the hepatitis-negative LCBs were more spread out ( Fig. 2f and Supplementary Fig. 5 ). This result indicates that chronic inflammation involved with hepatitis strongly influences the somatic substitution pattern ( Fig. 2e, f ). In addition, the substitution pattern of the hepatitis-negative LCBs was more similar to the recently reported ICCs [18] . To identify the mutational signatures of the hepatitis-positive or -negative LCBs, we used EMu software [27] for the 30 LCBs, and five mutational signatures were detected ( Supplementary Fig. 6 and 7 ). In these signatures, the influence of signature E, which consists of C>T mutations in CpG sites, differed significantly between the hepatitis-positive and -negative LCBs, indicating a potential role for methylated cytosines in carcinogenesis related with chronic hepatitis because C>T transitions preferentially occur in methylated CpG sites ( Supplementary Fig. 8 ). These findings suggest that the pattern of expressed genes is mainly influenced by cancer type and reflects histological or morphological classification, whereas the somatic substitution pattern in the LCBs is strongly determined by the aetiological background of chronic hepatitis. Recurrently mutated genes and pathway analysis We examined recurrently mutated genes in our LCB samples. RK308 had an exceptionally large number of mutations and was excluded from the subsequent analyses. Across the 29 LCB genomes, we detected 892 protein-altering mutations, including 760 nonsynonymous, 108 short coding indels and 24 splice-site mutations ( Supplementary Table 3 ). Thirty-two genes were recurrently mutated ( Fig. 3 and Supplementary Table 5 ): cytoskeleton genes ( XIRP2, KIF2B and MYO10 ), a cell adhesion molecule ( CDH2 ), known tumour suppressors ( TP53, PTEN and BAP1 ), known oncogenes ( KRAS and PIK3CA ), chromatin regulators ( PBRM1, ARID1A and ARID2 ), which are highly mutated in HCC and other cancers [10] , [12] , neuron growth genes ( ODZ1, EPHA2 and PLCO ) and tyrosine kinase receptors ( ERBB4 and EPHA2 ). To validate the frequency of the mutations, the protein-coding exonic regions of recurrently mutated genes ( BAP1, CDH2, EPHA2, KIF2B, MGAT4C, ODZ1, PBRM1, PCLO, SYT1, ARID2 and XIRP2 ) were amplified in an additional 68 LCB samples ( Supplementary Table 6 ) and sequenced by the Illumina HiSeq2000 sequencer. In addition, as KRAS, IDH1, IDH2 and TERT promoter mutations were frequently observed in ICCs [28] , fluke-related ICCs [18] and HCCs [29] , we sequenced exons 2 and 3 of KRAS, exon 4 of IDH1 (codon 132), exon 4 of IDH2 (codon 172) and TERT promoter hotspots (chr5:1,295,228 and 1,295,250) in the additional 68 samples by Sanger sequencing. TERT promoter hotspots were also examined in the 30 WGS samples by Sanger sequencing owing to a low depth of coverage in the WGS. This validation experiment revealed that one TERT promoter hotspot (chr5:1,295,228) was mutated in 14 samples (15.2%), KRAS and PBRM1 in 7 samples (10.3%), ARID2 in 5 (7.4%) , BAP1 , PCLO and IDH1 in 4 (5.9%), ODZ1 in three (4.4%) and EPHA2 , SYT2 , CDH2 , XIRP2 and IDH2 in two samples (2.9%) ( Fig. 3 and Supplementary Table 7 ). In the ARID2 , PBRM1 and BAP1 genes, which encode chromatin regulators, an accumulation of loss-of-function mutations was observed, suggesting that they are likely to function as tumour suppressors in LCBs as well as HCCs [10] , [12] . As observed in previous HCC studies [10] , [12] , [13] , more than half of LCBs had somatic mutations and rearrangements accumulated in chromatin regulators ( Supplementary Fig. 8 ). Figure 3: Analysis of recurrently mutated genes in LCBs. Recurrently mutated genes in the 30 LCB WGS set and the 68 validation LCB set. Histological subtype of LCB: ICC; intrahepatic cholangiocarcinoma, cHCC/CC; combined hepatocellular-cholangiocarcinoma and CoCC; cholangiolocellular carcinoma. Liver fibrosis was determined according to the New Inuyama Classification (0~4). Liver fibrosis 0 indicates hepatitis-negative LCB. Virus infection status is classified as HBV, HCV or negative, which was determined by serological study. Full size image We then examined the frequency of gene mutation and its association with clinical information in the WGS and validation samples ( Table 2 and Supplementary Table 8 ). The frequency of the TERT promoter hotspot mutations was significantly lower in LCBs than in HCCs (Fisher’s exact test P -value=1.2 × 10 −9 ) ( Table 2 ). Furthermore, the frequency was significantly higher in cHCC/CCs and HCCs than in the ICCs (Fisher’s exact test ICCs versus cHCC/CC; P- value=6.5 × 10 −5 and ICCs versus HCC; P -value=2.1 × 10 −11 ), but no significant difference was observed between cHCC/CCs and HCCs ( Table 2 ). The frequency of mutations in the KRAS and IDH gene hotspots and PBRM1 was higher in the LCBs than in the HCCs (not significant after the Bonferroni correction) and no mutations were observed in the 60 HCCs. Table 2 Summary of mutations in WGS and validation set of LCBs. Full size table When taking into account the presence of hepatitis, we found significant difference in the frequency of the TERT promoter hotspot mutations among the hepatitis-positive LCBs, the hepatitis-negative LCBs and the HCCs. The HCCs and hepatitis-positive LCBs had a higher frequency of the TERT promoter mutations than the hepatitis-negative LCBs ( Table 2 ). In contrast, HCCs had significantly lower frequency of KRAS and IDH gene hotspot mutations than the hepatitis-negative LCBs, all of which are ICCs (Fisher’s exact test KRAS ; P- value=0.0006, IDH genes; P -value=0.0006). Hepatitis-positive LCBs shared more mutated genes with HCCs, which is consistent with the substitution pattern shown in Fig. 2f . However, the frequency of mutations in the PBRM1 gene was different between hepatitis-positive LCBs and HCCs, which may be related to cell differentiation in the liver cancer development [30] (marginal significance after the Bonferroni correction). Mutations in the KRAS gene were significantly enriched in patients with lymph node metastasis ( Supplementary Table 8 ), and mutations in the BAP1 gene were significantly enriched in patients with vascular or bile duct invasion ( Supplementary Table 8 ). Mutations in IDH genes were associated with poor disease-free survival after adjustment for age, which is consistent with the previous study [20] ( Supplementary Fig. 10 ). To identify gene sets and pathways related to the LCB development, we carried out gene set enrichment analysis for all nonsynonymous mutations, short indels and rearrangements [31] . After adjustment for the multiple testing, 36 categories including ‘synapse organization’ and ‘cytoskeleton’ were significantly overrepresented ( Supplementary Table 9 ). These results suggest that genes in these categories have an important role in the carcinogenesis or cancer development in the LCBs. As ‘axon guidance’ genes were significantly mutated in pancreatic cancer [32] , genes related to neuron growth may have an important role in the carcinogenesis and development of aggressive hepato-biliary-pancreatic cancers, including LCBs. To determine any possible biological activity of these mutated genes in LCBs, we examined four genes ( PCLO , EPHA2 , ODZ1 and XIRP2 ), which are involved in synapse organization and/or cytoskeleton structure. We knocked down the expression of each candidate gene by short interfering RNA in liver cancer cell lines, and examined their proliferation, migration and invasion abilities. These experiments confirmed that silencing of PCLO promoted cell invasion in liver cancer cell lines ( Supplementary Figs 11 and 12 ). Genetic heterogeneity within liver tumour A tumour is a population of heterogeneous cancer cells, and the analysis of this heterogeneity should provide us with deeper insights into tumorigenesis [12] , [33] , [34] , [35] , [36] . To examine intratumour heterogeneity, the clonal proportion of the 1,085 nonsynonymous point mutations and short indels, detected in randomly selected 15 LCBs and 10 HCCs, were sequenced to an average depth of 56,462x by ultra-deep sequencing ( Supplementary Methods ). Copy number alternations were adjusted for mutant-allele frequencies using allelic imbalance ratio, and proportion of mutated allele (PMA) was obtained. The distribution of PMA in the ICCs and the cHCC/CCs significantly differed (Wilcoxon’s test P- value=0.0047), and ICC genomes had a larger number of mutations with higher PMA ( Supplementary Fig. 13 ). One possible explanation is that the pattern of genetic heterogeneity is different between cHCC/CC and ICC, and cHCC/CC had larger number of shared mutations in the tumour population than ICC, which is consistent with the histological diversity of cHCC/CC, showing mixed components of both hepatocellular and biliary epithelial differentiation. We then examined the clonal proportion for each gene ( Supplementary Dataset 2 ). Genes in 15 categories, including ‘replicative senescence’ and ‘negative regulation of DNA replication’ had a higher PMAs after adjustment for multiple testing ( Supplementary Table 10 ). All categories contained the TP53 gene, indicating that the TP53 gene conferred clonal advantage to cancer cells. This result is consistent with a breast cancer study [33] . Various genes showed high frequency of mutations in each tumour and would be candidates for tumour initiators ( Supplementary Dataset 2 ). In the present study, we comprehensively analyzed 30 LCBs by WGS and RNA-seq, and compared their genomic landscapes with those of 60 HCCs. To our knowledge, this is the first study that demonstrates the impact of chronic hepatitis and inflammation on the mutational landscape of the cancer genome and the first whole-genome comparison between LCBs and HCCs. In our analysis, gene expression patterns are consistent with the histological classifications; HCCs and LCBs were differentially clustered and hepatitis-positive and -negative LCBs were clustered together. In contrast, hepatitis-positive and -negative LCBs differentiated in their genome-wide somatic substitution pattern. The hepatitis-positive LCBs clustered more tightly to hepatitis-related HCCs, whereas hepatitis-negative LCBs were more spread out. These results suggest that gene expression depends on the histological phenotype, whereas the somatic substitution pattern is strongly influenced by aetiological background like the occurrence of chronic hepatitis. Previous studies suggested that the expression pattern is consistent with pathological phenotype, but does not reflect tumour origin [37] , [38] , [39] . A mouse study on pancreatic ductal adenocarcinoma suggested that inflammation can promote neoplasia by altering cell differentiation [38] , and a comparison between virus-associated ICCs and HCCs suggested that they can arise from the hepatic progenitor cells [5] . Considering these studies, the similarities between the hepatitis-positive LCBs and the HCCs in the somatic substitution pattern may indicate their same cellular origin, such as liver progenitor cell. In contrast, hepatitis-negative LCB may arise from different origins, such as cholangiocytes [40] . The frequency of some driver mutations, such as hotspot mutations in KRAS, IDH1/2 and TERT promoter, differed among cancer types, hepatitis-positive and -negative LCBs. Mutations of KRAS and IDH genes were more frequent in the hepatitis-negative LCBs, and the TERT promoter mutation was more frequent in the cHCC/CCs and HCCs. As almost all cHCC/CC and HCCs were hepatitis-positive, it is difficult to differentiate the impact of hepatitis from that of the histology. In general, HCC and cHCC/CC, which mainly developed under a hepatitis background, had a larger frequency of TERT promoter mutations and a lower frequency of KRAS and IDH1/2 mutations. In the current study, we found that the occurrence of chronic hepatitis impacted the mutational landscape, discovered new driver gene and examined intratumour heterogeneity in the LCBs. Our analysis indicates that the WGS can reveal the impact of aetiological background on the genome-wide substitution pattern, and suggest that the WGS can contribute to molecular classification based on their aetiology. However, we did not find mutations in the driver gene candidates in about a half of the samples, suggesting that LCB is a highly heterogeneous cancer. Analysis of larger number of samples would be necessary for deeper understanding of LCB. Clinical samples The clinical and pathological features of 30 LCBs that were used in WGS analysis are in Table 1 . Our pathologists evaluated hematoxylin and eosin-stained slides and diagnosed HCC, ICC and cHCC/CC according to the 2010 WHO Classification of Tumors of the Digestive System [41] . We defined ICC and cHCC/CC, both of which contain varying degrees of epithelial tubular-differentiated cells ( Fig. 1a ), as liver cancer displaying biliary phenotype (LCB), distinguishing them from the hepatocellular phenotype (HCC). Viral infection was defined by the presence of HB surface antigen in patient’s serum, or by the presence of antibody to HCV in patient’s serum. Hepatitis-negative LCB was defined as a tumour showing no sign of chronic inflammation and liver fibrosis, which was determined according the New Inuyama Classification. All subjects had undergone partial hepatectomy, and pathologists estimated the ratio of viable tumour cells in each sample. High molecular weight genomic DNA was extracted from fresh-frozen tumour specimens and blood. Non-cancerous liver tissues were used as the normal tissue for RK182, RK307, RK308, RK309 and RK310. All subjects agreed with informed consent to participate in the study following ICGC guidelines [42] . IRBs at RIKEN and all groups participating in this study approved this work. Whole-genome sequencing DNA was extracted from tumours and non-cancer frozen tissues, and 500 bp insert libraries were prepared according to the protocol provided by Illumina. The libraries were sequenced on HiSeq2000 platforms with paired reads of 101 bp. The mutation data for the 60 HCCs have been generated in the same way by RIKEN and deposited to the ICGC dataset version 8 released at 2012 March ( http://icgc.org/ ). Somatic mutation and short indel calling Point mutations and somatic indels were identified using our in-house methods [12] . In brief, read pairs were mapped by BWA [43] , and the result files were converted to pileup file by samtools [44] . After PCR duplications were removed and comparing between cancer genome sequences and non-cancer genome sequences, somatic point mutations and indels were identified by our in-house mutation caller [12] . False-negative and false-positive rates of our analysis pipeline were described previously [12] . Information for all point mutations and indels in the 30 LCBs and the 60 HCCs was deposited to the ICGC web site ( http://www.icgc.org/ ). Identification of rearrangements Inconsistent read pairs which occurred within 500 bp of each other were considered to support the same rearrangement. We identified candidate rearrangements in both tumour (support read pairs ≥4) and normal tissue (support read pairs ≥1) samples, and tumour-specific rearrangement candidates were identified. To exclude mapping errors, we performed a blast search of read pairs that support rearrangements against the reference genome. If a read pair mapped with correct orientation and distance (≤500 bp) with an E -value <10 −7 , we excluded that read pair. Reads mapped with more than two mismatches were also discarded. After filtering, candidates supported by ≥4 read pairs and at least one perfect match pair were considered as somatic rearrangements. The candidates that the same rearrangement was found in other normal samples were filtered out. False discovery rate of this method was estimated to be 2.3% (4/176). Statistical analysis The random distribution was calculated by multiplying (proportion of nucleotide in the reference genome sequence) and (total number of mutations) as done in the previous study [12] . Tests for significantly mutated genes and PCA of the substitution pattern were carried out as described previously [12] . Survival analyses were done using the ‘survival’ package for the R programming environment ( http://www.r-project.org ). A Cox proportional hazards model was used to test association between disease-free survival and mutations in the genes ( TERT promoter, KRAS , XIRP2 , ARID2 , BAP1 , PBRM1 , PCLO , ODZ1 and IDH genes) and clinical factors (age, gender, virus type and liver fibrosis). Model selection was done by the stepAIC function, and the model with age and mutations in IDH genes was selected. Estimation of PMA was described in the Supplementary Methods . To test the difference of the clonal proportion of mutations among ICCs, cHCC/CCs and HCCs, we calculated PMA for each mutation, which was standardized by the maximum PMA in each sample. Then we compared the median of the distribution of PMA between ICCs, cHCC/CCs and HCCs by Wilcoxon’s test. To identify gene sets with high clonal proportion, we used ‘biological process’ terms with depth=5 in the Gene Ontology (GO) database ( http://www.geneontology.org ). The clonal proportions of the genes within and outside the gene category were compared by Wilcoxon’s test as a previous study [33] . Note that we used unadjusted clonal proportions (not PMAs) for this analysis to consider the influence of copy number changes. Sanger sequencing and ultra-deep amplicon sequencing Sanger sequencing of PCR products was performed on ABI 3770x. For ultra-deep sequencing of mutations, each of the 100 bp target regions was amplified and the amplicons were directly ligated with Illumina TruSeq adaptors and sequenced on HiSeq2000 platform. Mapping was done by BWA to the target region, and uniquely mapped read pairs with proper distance and orientation were selected. More than 98% of the exonic target regions were covered with a depth ≥100. We filtered out reads with a mapping quality <10 and base calls with base quality <10. Base calls with a depth ≥100 were used for the analysis. We identified variants with frequency ≥0.05. Variants found in more than one individual in the 1000 Genome database [45] were discarded. We performed Sanger sequencing verification for the predicted candidates in the both cancer and matched normal tissues. RNA sequencing RNA-seq was carried out for 25 LCBs and 44 HCCs for which high-quality RNA was available among the 30 LCBs and the 60 HCCs. Total RNA was extracted by Trizol from the frozen liver cancer tissues and the corresponding non-cancerous liver tissues and quality and quantity were evaluated by Bioanalyzer (Agilent). The high-quality RNA was subjected to polyA+ selection and chemical fragmentation, and 100–200 base RNA fraction was used to construct complementary DNA libraries according to Illumina’s protocol. RNA-seq was performed on HiSeq2000 using the standard paired-end 101 bp protocol. Analysis of RNA sequencing data First, all sequencing reads were aligned to the known transcript sequences of UCSC known gene database ( http://hgdownload.cse.ucsc.edu/goldenPath/hg19/database/knownGene.txt.gz ) using Bowtie [46] , with -a --best --strata -m 20 -v 3 options, and the coordinates of the aligned reads were converted to the human reference sequence (hg19). Then, reads unaligned in the above step were aligned to the human reference sequence (hg19) and as well as HBV sequence (AP011098) using Blat [47] , with -stepSize=5 -repMatch=2253, and aligned reads by Bowtie or Blat were combined together. For each short read, the alignment positions with the maximum number of matched bases were adopted, and mapping quality for each read was assigned to as follows: for a location a , let B ( a ) denote the number of matched bases and let a best denote the best location selected arbitrarily from those with the maximum number of matched bases. Finally, sorting and PCR duplicate removal of short reads were performed by using Picard ( http://picard.sourceforge.net/ ). For quantification of expression values, we used a slightly modified version of RKPM (reads per kilobase of exon per million mapped reads) measures [48] . After removing improperly aligned or low-quality (mapping quality <60) sequencing reads, the number of bases on each exonic region for each refSeq genes ( http://hgdownload.cse.ucsc.edu/goldenPath/hg19/database/refGene.txt.gz ) were counted. Then, the numbers of bases were normalized as per kilobase of exon and per 100 million of aligned bases. Finally, the expression value of each gene was determined by choosing the maximum of multiple refSeq genes, if any, corresponding to the gene symbol. Accession codes: WGS data have been deposited in the EGA under the accession codes: EGAN00001187542, EGAN00001187543, EGAN00001187546, EGAN00001187547, EGAN00001187552, EGAN00001187553, EGAN00001187568, EGAN00001187569, EGAN00001187612, EGAN00001187613, EGAN00001187614, EGAN00001187615, EGAN00001187618, EGAN00001187619, EGAN00001187650, EGAN00001187651, EGAN00001187652, EGAN00001187653, EGAN00001187658, EGAN00001187659, EGAN00001187664, EGAN00001187665, EGAN00001187690, EGAN00001187691, EGAN00001187707, EGAN00001187708, EGAN00001187709, EGAN00001187710, EGAN00001187712, EGAN00001187713, EGAN00001187714, EGAN00001187715, EGAN00001187716, EGAN00001187717, EGAN00001187719, EGAN00001187720, EGAN00001187721, EGAN00001187722, EGAN00001187723, EGAN00001187724, EGAN00001187725, EGAN00001187726, EGAN00001187727, EGAN00001187728, EGAN00001187729, EGAN00001187730, EGAN00001187731, EGAN00001187732, EGAN00001187733, EGAN00001187734, EGAN00001187735, EGAN00001187736, EGAN00001187737, EGAN00001187738, EGAN00001187739, EGAN00001187740, EGAN00001187741, EGAN00001187742, EGAN00001187744 and EGAN00001187743 (summarized in Supplementary Table 2 ). How to cite this article: Fujimoto, A. et al. Whole-genome mutational landscape of liver cancers displaying biliary phenotype reveals hepatitis impact and molecular diversity. Nat. Commun. 6:6120 doi: 10.1038/ncomms7120 (2015).